Linkage control between molecular and supramolecular chirality in 21-helical hydrogen-bonded networks using achiral components Chiral molecules preferentially form one-handed supramolecular assemblies that reflect the absolute configuration of the molecules. Under specific conditions, however, the opposite-handed supramolecular assemblies are also obtained because of flexibility in the bond length and reversibility of non-covalent interactions. The mechanism of the handedness selectivity or switching phenomenon remains ambiguous, and most phenomena are observed by chance. Here we demonstrate the construction of chiral hydrogen-bonded twofold helical assemblies with controlled handedness in the crystalline state based on crystallographic studies. Detailed investigation of the obtained crystal structures enabled us to clarify the mechanism, and the handedness of the supramolecular chirality was successfully controlled by exploiting achiral factors. This study clearly reveals a connection between molecular chirality and supramolecular chirality in the crystalline state. The different levels of chirality linkage in materials have attracted much attention in the universal study of hierarchical structures [1] , [2] , [3] . On a molecular level, the linkage between monomers and macromolecules is evident in the handedness of helicity [4] , [5] , [6] , [7] , [8] . Chiral α-amino acids polymerize covalently to yield polypeptide chains involving helical conformations with right- or left-handedness that are indispensable for biomolecular function [9] , [10] , [11] . Alternatively, molecules assemble non-covalently to form helical supramolecules in the form of gels, liquid crystals and bulk crystals [12] , [13] . More than 70% of these crystals contain bundles of two-, three-, four- and/or sixfold helical assemblies that are characterized by mathematical space groups. However, the study of chirality linkages between molecules and the crystalline helical assemblies at the supramolecular level remains challenging. In general, the linkage can be expressed by a combination of two chiral centres producing two enantiomers and four diastereomers ( Fig. 1 ). A typical example of molecular chirality (MC) lies in the combination of two absolute configurations ( Fig. 1a ). In macromolecules, changes in handedness are evident in helicity ( Fig. 1b ). For example, polypeptide chains comprising L -amino acids primarily occur as right-handed α-helices, whereas special chains, such as poly( L -benzyl aspartate) form left-handed helices [14] . Similarly, MC may be connected to supramolecular chirality (SMC; Fig. 1c ). Helical hydrogen-bonding (HB) networks have become a target in the elucidation of the linkage between MC and SMC ( Fig. 1d ); organic molecules with ( R )- or ( S )-configurations produce two enantiomers and four diastereomers to form sup P or sup M helical HB networks. The symbols “ sup P ” or “ sup M ” represent the right- and left-handedness of the supramolecular helical assemblies [15] . The handedness control of these diastereomers may be based on subtle structural changes in the original molecules. 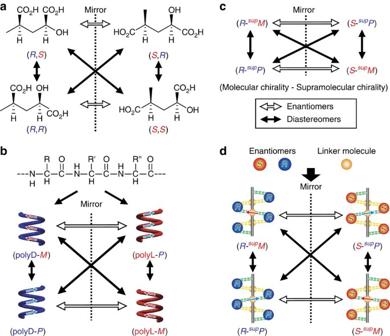Figure 1: Diastereomers with two different chiralities. (a) Conventional diastereomers resulting from two chiral carbons in molecular chirality. (b) Polymeric diastereomers with different molecular helicity. (c) Diastereomers with both molecular chirality and supramolecular chirality. (d) Supramolecular diastereomers with different supramolecular helicity for the 21-helical hydrogen-bonding networks. Figure 1: Diastereomers with two different chiralities. ( a ) Conventional diastereomers resulting from two chiral carbons in molecular chirality. ( b ) Polymeric diastereomers with different molecular helicity. ( c ) Diastereomers with both molecular chirality and supramolecular chirality. ( d ) Supramolecular diastereomers with different supramolecular helicity for the 2 1 -helical hydrogen-bonding networks. Full size image According to the Cambridge Structural Database, over 70% of organic crystals involve twofold (2 1 ) helical assemblies (see Supplementary Fig. S1 ) ( http://www.ccdc.cam.ac.uk/products/csd/statistics/ ). When studying steroidal inclusion crystals, we encountered a handedness problem with the 2 1 -helical assemblies of benzene molecules in channels and proposed a general concept (that is, supramolecular tilt chirality) to determine the handedness of the 2 1 -helices [16] , [17] . The discrimination method was further applied to the 2 1 -helices of HB networks of ammonium carboxylates [18] and Cinchona alkaloid derivatives [19] , as well as other 2 1 -helices [20] , [21] , [22] . These studies suggested a possible linkage control between MC and SMC, prompting us to investigate the flexible handedness control of the 2 1 -helices as shown in Fig. 1d . Herein we report the first example of linkage control of 2 1 -helical HB networks. We focus on the control of their diastereomers with achiral components and present a plausible mechanism for the inversion of the SMC of HB helices. Crystallographic studies and chirality analysis We employed chiral organic salts, A - or B -salts, composed of ( R )- or ( S )-α-methylbenzylamine (that is, A or B , respectively) with benzoic acid derivatives ( 1 – 5 ) ( Fig. 2a ). Crystallographic studies of the crystals, which were recrystallized from the salts, revealed that all of the crystals contained 2 1 -helical columns with one-dimensional (1D) ladder-type HB networks [18] , [23] . The charge-assisted hydrogen bonds between the amines and carboxylic acids have a length of 2.71–2.83 Å (see Supplementary Table S1 ). In addition, the crystals were subjected to powder X-ray diffraction (PXRD) analysis. The resulting peak patterns coincided with those calculated from the single-crystal X-ray analysis data (see Supplementary Figs S2 and S3 and Supplementary Tables S2 to S5 ). On the basis of these results, the diastereomers of the crystals do not exhibit polymorphic forms, with the exception of crystals formed from p -chloro- or p -bromobenzoic acid. 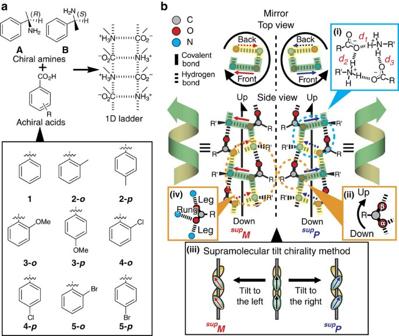Figure 2: Helicity and handedness of one-dimensional ladder-type hydrogen-bonding networks. (a) Primary ammonium carboxylates employed in this study. The organic salts are composed of chiral amineAorBwith achiral benzoic acid derivatives (1–5). (b) Twofold helical hydrogen-bonding networks with repetition of deformed rings (inset (i)) based on discriminableO(α) andO(β) of carboxylate groups (inset (ii)). Right or left handedness are determined according to the supramolecular tilt chirality method (inset (iii)) and referred to assupPorsupM, respectively. The rung N–O(α) portion (inset (iv)) is located on the front and back sides in the top views, which are indicated in green and yellow, respectively. The right or left tilt of the rung portions on the front sides defines the right- or left-handedness of the 21-helices (inset (iii)). The upward direction of the networks is defined along the direction ofO(α) toO(β) on the leg portions (inset (ii)). Figure 2: Helicity and handedness of one-dimensional ladder-type hydrogen-bonding networks. ( a ) Primary ammonium carboxylates employed in this study. The organic salts are composed of chiral amine A or B with achiral benzoic acid derivatives ( 1 – 5 ). ( b ) Twofold helical hydrogen-bonding networks with repetition of deformed rings (inset (i)) based on discriminable O (α) and O (β) of carboxylate groups (inset (ii)). Right or left handedness are determined according to the supramolecular tilt chirality method (inset (iii)) and referred to as sup P or sup M , respectively. The rung N– O (α) portion (inset (iv)) is located on the front and back sides in the top views, which are indicated in green and yellow, respectively. The right or left tilt of the rung portions on the front sides defines the right- or left-handedness of the 2 1 -helices (inset (iii)). The upward direction of the networks is defined along the direction of O (α) to O (β) on the leg portions (inset (ii)). Full size image All the resulting single crystals belong to chiral space groups and have 1D ladder-type HB networks with 2 1 -helicity. The handedness of the 2 1 -helicity was determined using the supramolecular tilt chirality method ( Fig. 2b , inset (iii)) and is listed in Table 1 , where right- or left-handedness of the SMC is symbolized as sup P or sup M , respectively, along with absolute configurations (that is, R and S ) of the amines. First, we ascertained the usual enantiomeric relationship of the helical HB networks using A - and B -salts with methylbenzoic acid ( 2 ). The crystals of A(2- o ) and B(2- o ) belong to the monoclinic C 2 space group. A(2- o ) with ( R )-isomers display R - sup P , whereas B(2- o ) with ( S )-isomers is S - sup M , as expected ( Fig. 3a (i)). Non - and para -substituted acids introduced a drastic change; the crystals of A(1) and A(2- p ) belong to the orthorhombic P 2 1 2 1 2 1 space group and are R - sup M , in contrast to the R - sup P structure of A(2- o ) ( Fig. 3a (ii)). This pair of supramolecules can be regarded as pseudo-diastereomers. Table 1 Crystal parameters of the salts. 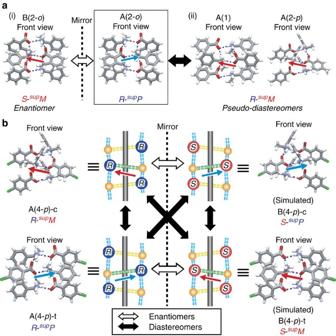Figure 3: Enantiomeric and diastereomeric linkages between molecular chirality and supramolecular chirality. (a, i) Enantiomeric linkage in the hydrogen-bonding networks ofA(2-o)–B(2-o), and (ii) pseudo-diastereomeric linkage in the hydrogen-bonding networks ofA(2-o)–A(1)andA(2-o)–A(2-p). (b) Enantiomeric and diastereomeric linkages in the hydrogen-bonding networks ofA(4-p)-c,A(4-p)-t,B(4-p)-candB(4-p)-t, in which four diastereomeric linkages between molecular chirality and supramolecular chirality are observed. Full size table Figure 3: Enantiomeric and diastereomeric linkages between molecular chirality and supramolecular chirality. ( a , i) Enantiomeric linkage in the hydrogen-bonding networks of A(2- o )– B(2- o ), and (ii) pseudo-diastereomeric linkage in the hydrogen-bonding networks of A(2- o )– A(1) and A(2- o )– A(2- p ). ( b ) Enantiomeric and diastereomeric linkages in the hydrogen-bonding networks of A(4- p )-c , A(4- p )-t , B(4- p )-c and B(4- p )-t , in which four diastereomeric linkages between molecular chirality and supramolecular chirality are observed. Full size image This result prompted us to employ other substituents, such as methoxy, chloro and bromo groups, with A -salts with ( R )-configurations. Table 1 shows that the salts with the para -substituted or ortho -substituted acids are R - sup M or R - sup P , respectively. Surprisingly, the A(4- p ) and A(5- p ) salts formed both R - sup M crystals and R - sup P crystals as polymorphs, indicating the formation of a pair of true diastereomers. The result suggests four types of diastereomeric relationships between MC and SMC ( Fig. 3b ), as theoretically expected ( Fig. 1d ). In other words, the HB helices exhibit a stereoisomeric relationship similar to the covalently bonded helices. To the best of our knowledge, this is the first example of the existence of diastereomers with a linkage between the absolute configurations of the molecules and the helical conformations with hydrogen bonds in the crystalline state. In addition, these results clearly indicate that achiral components can control the linkage between MC and SMC in crystals. Measurements of vibrational circular dichroism spectra To further confirm the handedness switching of the SMC of the HB networks, solid-state vibrational circular dichroism (VCD) spectra and infrared spectra were measured for the A(4- p ) crystal with a chirality of R - sup M , R - sup P and the B(4- p ) crystal, with a chirality of S - sup P , S - sup M , which are denoted as A(4- p )-c , A(4- p )-t and B(4- p )-c , B(4- p )-t , respectively, using KBr pellets ( Fig. 4 ). The terminal symbols - c and - t represent the coplanar and twisted conformations, respectively, of the carboxylic groups relative to the phenyl rings. The chiral properties can be measured using VCD spectra instead of electronic circular dichroism spectra, because the handedness of the SMC was defined by the HB networks between the amino and carboxylic groups, which have specific absorptions in the infrared region. The infrared spectra are nearly identical in all of the cases. For the VCD signals, a mirror-image relationship is observed between the enantiomeric pairs of A(4- p )-c and B(4- p )-c ( Fig. 4a ), as well as in A(4- p )-t and B(4- p )-t ( Fig. 4b ), confirming the reliability of the signals. The most discriminative VCD signals are at ~1,530 (number 1–3 in the figure) and 1,380 cm −1 (number 4–6), and inversion of the signals is clearly observed in the VCD signals of the diastereomeric pairs of A(4- p )-c and A(4- p )-t , as well as of B(4- p )-c and B(4- p )-t . This result strongly supports the handedness switching of the SMC of the HB networks. 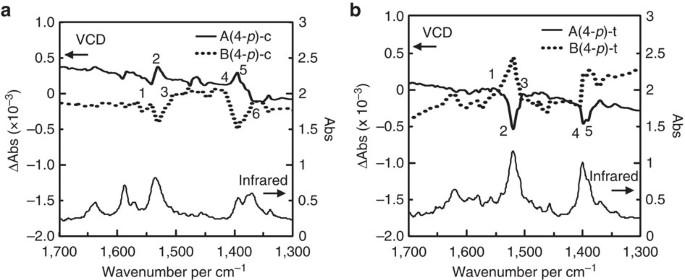Figure 4: Solid-state vibrational circular dichroism spectra. (a) The vibrational circular dichroism spectra ofA(4-p)-candB(4-p)-cand (b)A(4-p)-tandB(4-p)-t; the spectra of theA-salts andB-salts are represented by solid and dotted lines, respectively. Figure 4: Solid-state vibrational circular dichroism spectra. ( a ) The vibrational circular dichroism spectra of A(4- p )-c and B(4- p )-c and ( b ) A(4- p )-t and B(4- p )-t ; the spectra of the A -salts and B -salts are represented by solid and dotted lines, respectively. Full size image The reliability and the origins of the observed signals were also confirmed by density functional theory calculations of the HB networks of the salts of A(4- p )-c and A(4- p )-t . VCD calculations were performed for HB columns composed of five amines and five carboxylic acids (not merely the ion pair of one amine and one acid), because the assembly manner is important for the generation of SMC. The geometry optimizations did not substantially change the geometries of the columns. The calculation conditions and calculated spectra are shown in the Supplementary Information (see Supplementary Fig. S4 ). The optimized columnar structures are strained compared with the observed structures. However, their handedness is still distinguishable because of the robust charge-assisted HBs and, therefore, the calculated VCD signals are in good agreement with the observed signals, with the exception of the spectral shifts. According to the calculation, the signals at ~1,530 cm −1 (number 1–3; calculated to be ~1,640 cm −1 ) primarily correspond to stretching of the C–O of the carboxylic groups and bending of the N–H of the amino groups. The signals at ~1,380 cm −1 (number 4–6) (calculated to be ~1,440 cm −1 ) primarily correspond to stretching of the C–C between the carboxylic groups and adjacent α-carbons and bending of the C–H of the methyl groups of the amines. Thus, the functional groups that form the HB networks and the other moieties around the HB networks are related to the handedness of the SMC. Handedness switching mechanism The handedness switching of the SMC, which is a function of its substituents, corresponds to asymmetry generation, which is linked to MC. To clarify the switching mechanism, we compared three aspects of the detailed crystal structures: (i) tilt of the carboxylate group compared with the helical axis, (ii) conformations of the carboxylate group compared with the linked phenyl ring and (iii) herringbone stacking of the phenyl rings. 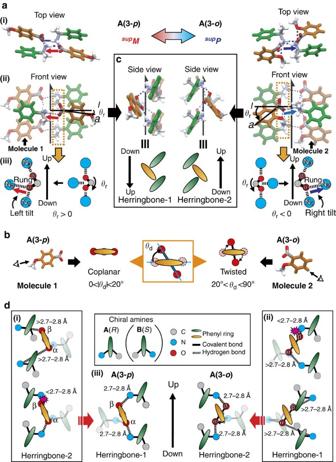Figure 5: Possible mechanism of handedness switching. (a) (i) Top views, (ii) front views and (iii) positions of the carboxylic groups relative to the amino groups with rotation angles,θr, of the hydrogen-bonding 21-helical columns ofA(3-p) (left) andA(3-o) (right) with supramolecular chiralities ofsupMandsupP, respectively. (b) Two types of conformation ofA(3-p) (left) andA(3-o) (right) with dihedral angles,θd. (c) Side views of the hydrogen-bonding 21-helical columns ofA(3-p) (left) andA(3-o) (right); up and down are defined from concave to convex of the herringbone assemblies of the phenyl rings. The direction of herringbone-1 is the opposite of that of the hydrogen-bonding networks whereas that of herringbone-2 is the same. (d) A mechanism for the selected formation of herringbone-1 inA(3-p) (left) and herringbone-2 inA(3-o) (right). The length of the hydrogen bonds are unfavourable for (i) herringbone-2 and (ii) herringbone-1 inA(3-p) andA(3-o), respectively, and (iii) favourable for herringbone-1 and herringbone-2 inA(3-p) andA(3-o), respectively. Figure 5 exemplifies the comparative structures of a pair of A(3- p ) and A(3- o ), where the same amines with ( R )-configurations yield reverse HB networks with sup M and sup P due to the para - and ortho -methoxy groups, respectively. Figure 5: Possible mechanism of handedness switching. ( a ) (i) Top views, (ii) front views and (iii) positions of the carboxylic groups relative to the amino groups with rotation angles, θ r , of the hydrogen-bonding 2 1 -helical columns of A(3- p ) (left) and A(3- o ) (right) with supramolecular chiralities of sup M and sup P , respectively. ( b ) Two types of conformation of A(3- p ) (left) and A(3- o ) (right) with dihedral angles, θ d . ( c ) Side views of the hydrogen-bonding 2 1 -helical columns of A(3- p ) (left) and A(3- o ) (right); up and down are defined from concave to convex of the herringbone assemblies of the phenyl rings. The direction of herringbone-1 is the opposite of that of the hydrogen-bonding networks whereas that of herringbone-2 is the same. ( d ) A mechanism for the selected formation of herringbone-1 in A(3- p ) (left) and herringbone-2 in A(3- o ) (right). The length of the hydrogen bonds are unfavourable for (i) herringbone-2 and (ii) herringbone-1 in A(3- p ) and A(3- o ), respectively, and (iii) favourable for herringbone-1 and herringbone-2 in A(3- p ) and A(3- o ), respectively. Full size image First, the deformation of the network provides evidence for the tilt generation. Figure 5a(i display top- and front views of the 2 1 -helical HB network, respectively. Starting from a geometrically symmetric position ( Fig. 5a (iii)), the carboxylate group rotates clockwise or anticlockwise to yield the distinguishable oxygen atoms (that is, O (α) with two HBs and O (β) with one HB) due to the restriction of the HB length ( d 1 , d 2 , d 3 are ~2.7 to 2.8 Å, Fig. 2b inset (i) and see Supplementary Table S1 ). The different oxygen atoms enable us to discriminate two directions, including up and down, as well as right and left ( Fig. 2b (ii, iii, iv) and Fig. 5a (iii)). The upward direction is defined from N 1 through O (α) and O (β) to N 3 along the leg linkage, whereas the right and left direction is defined from the O (α)–N 2 linkage of the rung portion. The resulting asymmetric network is described below. The ( sup M )-network of A(3- p ) ( Fig. 5a , left) has a carboxylate group at the front and right side. Clockwise rotation of the group yields the left tilt (upward to left) of the rung O (α)–N part. The rotation angle ( θ r ; Fig. 5a (iii)) is evaluated based on the tilt of the linked phenyl ring from the horizontal line. The tilt angle from the helical axis corresponds to (90+ θ r ). The ( sup P )-network of A(3- o ) ( Fig. 5a , right) exhibits anticlockwise rotation of the carboxylate on the front and left side to yield the right-tilt with the tilt angle (−(90– θ r )). Second, a notable difference lies in the conformations between the carboxylate group and the linked phenyl ring. From Fig. 5b , the ( sup M )-network of A(3- p ) has a coplanar conformation, whereas the ( sup P )-network of A(3- o ) has a twisted one. The dihedral angles ( θ d ) are listed in Table 1 . Coplanar conformations are observed for benzoic acid and its p -substituted derivatives, whereas twisted conformations are observed for o -substituted derivatives of benzoic acid. This handedness switching due to o -substitution is attributed to steric repulsion between the carboxylate group and the o -substituent. Indeed, the carboxylate group with the coplanar conformation experiences repulsion from the methoxy group due to the close contact. Third, we observed a herringbone stacking of phenyl rings in the right- or left-side view. The herringbone stacking has a concave and a convex component, enabling us to define its up and down direction. The upward direction is defined from the convex to the concave component along the helical axis. From Fig. 5c , the direction of A(3- p ) is the reverse of that of A(3- o ). As the HB networks have the same direction for both cases, the coplanar conformation has an inverse direction between the HB networks and herringbone stacking (herringbone-1), whereas the twisted conformation has the same direction (herringbone-2). From the abovementioned three viewpoints, the mechanism of the handedness switching is considered to be as follows. Figure 5d shows a carboxylic acid molecule surrounded by one amine molecule on the rung portion and two amine molecules on the leg portion. The phenyl ring of the acid molecules exhibits a left tilt in both A(3- p ) and A(3- o ). The amine molecules on the leg and rung portions are located on the right- and left side of herringbone-1 of A(3- p ), respectively, whereas the locations of these amine molecules are inverted in herringbone-2 of A(3- o ). Therefore, the amine molecules with ( R )-configurations exhibit two types of herringbone-1 and -2, and the twisted conformation introduces an exchange to herringbone-2 from herringbone-1. Instead of herringbone-2, the twisted conformation may exhibit herringbone-1, which is unfavourable because of restrictions from the length of the HB bonds for the 1D helical network. In conclusion, this study demonstrates the handedness switching of SMC of 1D ladder-type HB networks based on the twist of carboxylate groups with o -substituents on the achiral carboxylic acids due to steric repulsion. To the best of our knowledge, this is the first demonstration of handedness switching of SMC by achiral counter ions, and we have confirmed the switching based on crystal structures as well as VCD spectra. Although chiral molecules preferentially construct one-handed superstructures reflecting MC, including in biomolecules such as proteins and DNA, the mechanism remains unclear. This crystalline system demonstrated a connection between MC and SMC. In addition, the VCD spectra clearly reflected the handedness switching of helices composed of ammonium carboxylates clarifying this correlation. Therefore, this work has the potential to clarify important features of small molecules as well as proteins via VCD studies [24] . Further study is now underway to define the properties resulting from SMC switching and selective molecular assembly in specific space groups. Crystallographic study The corresponding amine and acid were mixed in methanol followed by evaporation in vacuo to yield powdered salts. Then, the salts were recrystallized from chloroform/hexane or ethanol/toluene mixed solution to afford single crystals that were suitable for X-ray analysis. Single-crystal X-ray diffraction data were collected on a Rigaku RAXIS-RAPID imaging plate diffractometer with graphite-monochromated CuKα radiation ( λ =1.54187 Å), with the exception of A(2- p ), for which data were collected using synchrotron radiation ( λ =0.8000 Å) at the BL38B1 in the SPring-8 synchrotron radiation facility. Cell refinements were performed with HKL2000 software [25] for A(2- p ). The lattice parameters were obtained by least-square analysis of the reflections for three oscillation images. The structure solution was achieved by direct methods using SIR2004 or SHELXS97 ( [26] , [27] ). The structures were refined using a full matrix least-square procedure, with all of the observed reflections based on F [2] . All of the non-hydrogen atoms were refined with anisotropic displacement parameters, and the hydrogen atoms were placed in idealized positions with isotropic displacement parameters relative to the connected non-hydrogen atoms and were not refined. All of the calculations were performed with the CrystalStructure crystallographic software package [28] , with the exception of the refinement, which was performed using the SHELXL-97 programme. The crystallographic data for this study have been deposited at the Cambridge Crystallographic Data Centre. Their crystallographic parameters are provided in the Supplementary Information . PXRD data were collected on the powdered salts, which were prepared by grinding the crystals, with a Rigaku RINT-2000 diffractometer using graphite-monochromatized CuKα radiation ( λ =1.54187 Å) at room temperature. Solid-state VCD spectra The VCD and infrared spectra of the solid states were measured with a PRESTO-S-2007 spectrometer (JASCO, Co., Japan) using KBr pellets. The machine is a single photoelastic modulator system, and the central wavenumber of photoelastic modulator was set at 1,250 cm −1 . The calibration was performed using of a quarter wave retardation and an analyser. The crystals of A(4- p )-c and A(4- p )-t were prepared from the chloroform solution of the salt of A(4- p ) by rapid cooling and slow evaporation. The crystals of B(4- p )-c and B(4- p )-t were obtained using the same method. The purities of the crystals were determined by PXRD analysis. A KBr pellet of each crystal was injected into an assembled cell with a window of 5 mm φ . The signal was accumulated during 5,000 scans ( ca . 1 h) for each crystals. The resolution was 4 cm −1 . The absorbance of the infrared spectra was adjusted to ~1 for optimal measurements. The measurements were also conducted after rotating or reversing the KBr pellets to confirm the reliabilities of the signals accumulated during 2,000 scans ( ca . 0.5 h). Computational details The theoretical infrared and VCD spectra of the salts of A(4- p )-c and A(4- p )-t were calculated using the Gaussian 09 programme [29] , [30] . The initial 1D columnar structures, which consisted of five amines and five carboxylic acids, were extracted from the crystal structures of the salts. Their phenyl and p -chlorophenyl groups were replaced with methyl groups to conserve computer time. The geometry optimizations and VCD calculations were performed using density functional theory at the B3LYP/6-31G ( d , p ) level of theory. The observed spectra were assigned based on animations of the molecular vibration with Gauss View 5.08 software (Gaussian Inc.) [31] . Accession codes: The X-ray crystallographic coordinates for structures reported in this Article have been deposited at the Cambridge Crystallographic Data Centre (CCDC), under deposition numbers CCDC 898257, 898260, 898267, 898265, 898261, 898266, 898259, 898264, 898258, 898262 and 898263 for A(1) , A(2- o ), B(2- o ), A(2- p ), A(3- o ), A(3- p ), A(4- o ), A(4- p )-t , A(5- o ), A(5- p )-c and A(5- p )-t , respectively. These data can be obtained free of charge from The Cambridge Crystallographic Data Centre via www.ccdc.cam.ac.uk/data_request/cif . How to cite this article: Sasaki, T. et al . Linkage control between molecular and supramolecular chirality in 2 1 -helical hydrogen-bonded networks using achiral components. Nat. Commun. 4:1787 doi: 10.1038/ncomms2756 (2013).